Negative refraction of elastic waves at the deep-subwavelength scale in a single-phase metamaterial Negative refraction of elastic waves has been studied and experimentally demonstrated in three- and two-dimensional phononic crystals, but Bragg scattering is impractical for low-frequency wave control because of the need to scale the structures to manageable sizes. Here we present an elastic metamaterial with chiral microstructure made of a single-phase solid material that aims to achieve subwavelength negative refraction of elastic waves. Both negative effective mass density and modulus are observed owing to simultaneous translational and rotational resonances. We experimentally demonstrate negative refraction of the longitudinal elastic wave at the deep-subwavelength scale in the metamaterial fabricated in a stainless steel plate. The experimental measurements are in good agreement with numerical simulations. Moreover, wave mode conversion related with negative refraction is revealed and discussed. The proposed elastic metamaterial may thus be used as a flat lens for elastic wave focusing. Negative refraction (NR) was first proposed as a theoretical possibility in electromagnetic waves [1] and promises exciting avenues to various applications such as super-resolution imaging to overcome diffraction limit [2] , [3] , [4] . Two types of NR have been intensively studied. The first uses electromagnetic metamaterials with simultaneous negative permittivity and negative permeability [5] , while the second arises from photonic crystals with an effective refractive index controlled by the band structure [6] . On the basis of the acoustic analogues of photonic crystals, NR of acoustic waves has been theoretically and experimentally demonstrated by carefully tailoring the dispersion band in the Brillouin zone of phononic crystals (PCs). Yang et al. [7] experimentally achieved NR and focusing of ultrasound beams by using the anisotropy of the equifrequency curves (EFCs) in a PC consisting of tungsten carbide beads surrounded by water. NR imaging for all angles of incidence was demonstrated later through the EFCs in the second band of a two-dimensional (2D) PC, where the direction of the wave vector and group velocity are antiparallel to each other [8] , [9] , [10] . Intense Bragg scattering at the Brillouin zone can also result in the extreme deformation of the second band EFCs in PCs, which leads to backward-wave NR [11] . Subwavelength imaging has been demonstrated experimentally with PCs [12] and super-resolution of a PC flat lens has been achieved by resonantly amplifying evanescent waves [13] . More recently, Christensen et al. [14] , [15] proposed a holey anisotropic metamaterial to obtain subwavelength NR and focusing by using the hyperbolic dispersion of a sound wave. The dependence of the band structure on periodically arranged unit cells usually limits the practical applications of PCs, often by requiring the size of the device to be the same order of magnitude as the acoustic wavelength. To overcome that, a locally resonant (LR) acoustic metamaterial has been developed to achieve subwavelength NR. At the subwavelength scale, effective medium theory shows that the metamaterial can possess simultaneous negative mass density and bulk modulus [16] , [17] , which lead to negative effective refractive index and subwavelength focusing [18] . He et al. [19] combined the LR units along with a water-immersed epoxy plate patterned with periodical heavy gratings to achieve negative index. Yang et al. [20] experimentally demonstrated a double-negative acoustic metamaterial with a single resonating structure. Although a large amount of research work has been reported on NR of acoustic waves in fluid-like media, relatively fewer experimental demonstrations exist on NR of elastic waves in solid media where the coupled longitudinal and transverse waves bring challenging but richer wave phenomena. All of the reported experiments on NR of elastic waves in solid bulk media are based on Bragg scattering. Using a unit cell size ≈ λ , NR of transverse and longitudinal waves was experimentally observed in 2D PCs made of cylindrical air cavities in an aluminium (Al) block at 470–530 kHz and steel rods embedded in an epoxy matrix at 750–860 kHz, respectively [21] , [22] . For elastic guided waves, Pierre et al. [23] employed a 2D PC with a unit cell size ≈2.7 λ and experimentally evidenced the NR of antisymmetric Lamb waves at 5.4–10.5 MHz. Lee et al. [24] conducted NR experiments with guided shear-horizontal waves in a thin PC plate with unit cell size ≈0.63 λ at 210–260 kHz. Dubois et al. [25] investigated elastic wave propagation in a thin PC plate with circular perforated air holes. The lattice constant is 0.34 λ at 10 kHz and the dispersion band is used to generate NR and achieve focusing. A NR of Lamb waves was demonstrated by conversion between forward- and backward-propagating modes at the interface where the plate thickness changes [26] . Elastic metamaterials (EMMs), on the other hand, have the capability to achieve unique and unprecedented effective elastic properties based on the local resonance mechanism. For isotropic EMMs, the three relevant effective properties are bulk modulus, shear modulus and mass density, the negative effective elastic parameters can be realized by promoting monopolar, dipolar and quadrupolar resonances with resonant microstructures into the building blocks of an EMM [27] , with the ultimate goal of attaining a negative index of refraction [28] , [29] . In these cases, the EMM can function as a left-handed medium, that is, S·k <0 where S represents the Poynting vector and k is the wave vector. In particular, Wu et al. [29] employed a fluid-solid microstructure and numerically studied the NR of a transverse wave in an EMM possessing both negative mass density and negative shear modulus. At the same time, an EMM made of three-phase solid media is numerically demonstrated to possess simultaneous negative mass density and negative bulk modulus by introducing a chirality [30] . However, for all existing designs, the constraints on the physical properties of the components are so severe that those approaches remain exploratory to a large extent. Because of this, no experimental demonstration of NR of elastic waves at the deep-subwavelength scale by using EMMs has been reported so far. In this article, we propose an EMM with chiral microstructure made of a single-phase material to experimentally demonstrate NR of elastic waves at the deep-subwavelength scale. The effective mass density and bulk modulus of the proposed EMM have simultaneous negative values owing to simultaneous translational and rotational resonances. NR of longitudinal incident elastic waves is demonstrated by using a prism-shaped EMM with unit cell size ≈0.1 λ fabricated in a stainless steel plate at 41.8–45.0 kHz. In the experiment, the longitudinal wave is excited by using symmetrically bonded piezoelectric patches and the refracted in-plane elastic waves are measured by using a 3D laser scanning vibrometer. The measured results are in excellent agreement with the numerical predictions. The experimental observation of the NR of elastic waves at the deep-subwavelength scale is the first step towards the construction of subwavelength elastic wave imaging devices. Finally, a wave mode separation analysis is systematically investigated to reveal the elastic wave mode conversion behaviour of the negatively refracted waves. Single-phase EMM for subwavelength NR The unit cell microstructural design of the EMM in a triangular array is shown in Fig. 1a , which is composed of a single-phase solid material. The unit cell of chiral microstructure is designed by properly slot cutting in a hexagonal area and forming three chirally distributed ribs to connect the centre piece (functioning as a mass) and the frame. The lattice constant is a , and widths of the slot, ribs and frames are s , r and t f , respectively. r f represents the radius of the fillet between the rib and the frame. In this design, the three ribs are critical since they will induce not only the translational resonance but also the rotational resonance to the centre piece, as shown in Fig. 1b,c , respectively. Therefore, by carefully selecting the dimension of the chirally distributed ribs, it is possible to achieve and enhance simultaneous translational and rotational resonances and NR at a desired low-frequency range. The wave mechanism of the EMM with chiral microstructure was interpreted and can be found in ref. 31 . 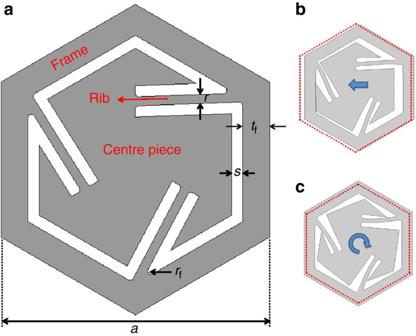Figure 1: Unit cell design of the EMM with chiral microstructure and its modes. (a) The unit cell of the single-phase EMM with chiral microstructure. (b) The mode of the translational resonance. (c) The mode of the rotational resonance. Figure 1: Unit cell design of the EMM with chiral microstructure and its modes. ( a ) The unit cell of the single-phase EMM with chiral microstructure. ( b ) The mode of the translational resonance. ( c ) The mode of the rotational resonance. Full size image Knowing the effective medium parameters of a metamaterial is very useful for efficiently studying its wave propagation characteristics. Due to the geometric complexity, the use of analytical methods to obtain effective properties of the proposed EMM with chiral microstructure is not practicable. Instead, a numerical-based effective medium method based on the micromechanics approach is adopted, which is under the long-wavelength assumption [32] . The effective medium theory links the microscopic resonant structures to the EMM’s macroscopic parameters. In the unit cell analysis, the global (macroscopic) stress, strain, resultant force and acceleration of the unit cell can be numerically calculated by averaging local quantities on the external boundary of the hexagonal cell. Then, on the basis of the constitutive relationship, the effective bulk modulus, shear modulus and mass density of the proposed EMM with chiral microstructure can be determined from the calculated macroquantities. On the basis of the numerical-based effective model, the effective bulk modulus and mass density of the EMM are calculated and shown in Fig. 2b,c , respectively. The effective mass density ρ eff and bulk modulus K eff are normalized with the density and Young’s modulus of the single-phase medium (stainless steel), respectively. The dispersion curves of the system along the ΓM direction are also numerically obtained based on the Floquet theory, as shown in Fig. 2a . The unit cell geometrical and material properties of the EMM are listed in Table 1 . 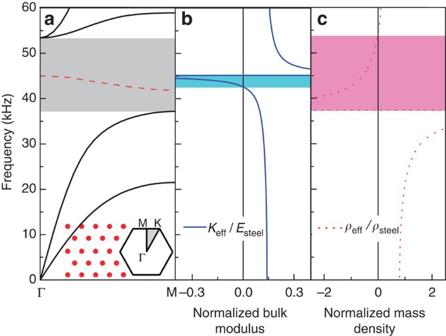Figure 2: Dispersion curves and effective material properties of the single-phase EMM. (a) Dispersion curves along ΓM direction (black solid lines) with highlighted negative pass band (red dashed line). The grey shaded region represents the bandgap and the inset shows the lattice array of the EMM and its irreducible Brillouin zone (IBZ). (b) Effective bulk modulus of the EMM (blue solid line). The blue shaded region highlights the frequency range of the negative effective bulk modulus. (c) Effective mass density of the EMM (red dotted line). The pink shaded region highlights the frequency range of the negative effective mass density. Figure 2: Dispersion curves and effective material properties of the single-phase EMM. ( a ) Dispersion curves along ΓM direction (black solid lines) with highlighted negative pass band (red dashed line). The grey shaded region represents the bandgap and the inset shows the lattice array of the EMM and its irreducible Brillouin zone (IBZ). ( b ) Effective bulk modulus of the EMM (blue solid line). The blue shaded region highlights the frequency range of the negative effective bulk modulus. ( c ) Effective mass density of the EMM (red dotted line). The pink shaded region highlights the frequency range of the negative effective mass density. Full size image Table 1 Unit cell geometrical and material parameters of the EMM with chiral microstructure. Full size table As evidenced in Fig. 2 , the frequency range of the bandgap predicted from the dispersion calculation (37.2–53.6 kHz) is almost the same as the frequency range with negative ρ eff (37.4–54.1 kHz) as shown in Fig. 2c , which can be explained by the out-of-phase translational motion of the centre piece against the frame. As shown in Fig. 2b , K eff becomes negative in the frequency range of 42.9–45.0 kHz. The effective shear modulus μ eff is calculated as 16.23 GPa in the considered frequency range with a small variation. Eventually, both effective longitudinal modulus E eff = K eff + μ eff and effective mass density ρ eff become negative in the region from 43.6 to 45.0 kHz, which implies a negative band for the longitudinal wave in this frequency region. It is also noticed that the double-negative frequency region (43.6–45.0 kHz) is not the same as the total negative passband frequency region (41.8–45.0 kHz) from the dispersion curves, as shown in Fig. 2a . The difference can be attributed to the strong anisotropy of the current microstructural design, which cannot be exactly captured by using the effective isotropic medium [31] . For the chiral topology, the number of the chirally distributed ribs, N r , is an important parameter for the global property of the EMM with chiral microstructure. The EMM becomes more isotropic when N r is a larger value, while displaying stronger anisotropy when N r is a smaller value. In the current design, the metamaterial tends to be anisotropic since there are only three ribs used, which is also reflected by the EFCs in non-perfect circular shapes that we will demonstrate later. Finally, it should also be mentioned that the longitudinal wavelength in the host medium at the negative passband frequency region is from 112 to 121 mm, which is much larger than the unit cell size of the microstructure that is 12 mm. Numerical simulation and experimental measurements Both numerical and experimental studies will be presented to illustrate the subwavelength NR by the proposed single-phase EMM with chiral microstructure. First, a transient wave propagation in a 30° prism-shaped EMM plate consisting of 256 EMM unit cells is simulated using commercial finite element software LS-DYNA, as shown in Fig. 3a . Absorbing boundaries are applied to the entire region to eliminate the boundary reflection. Displacement excitation along the horizontal direction ( x direction) is applied to the central part of the left side of the EMM prism to simulate a plane longitudinal wave incidence with the transverse width of 8.75 a . A 50-cycle tone burst is chosen to excite resonant motion around the central frequency f c . The waveform ( f c =43.8 kHz) and corresponding frequency spectrum are given in Fig. 3b . The frequency bandwidth of the tone-burst signal is 1.7 kHz (full width at half maximum), which makes it possible to evaluate wave propagation at the central frequency f c . 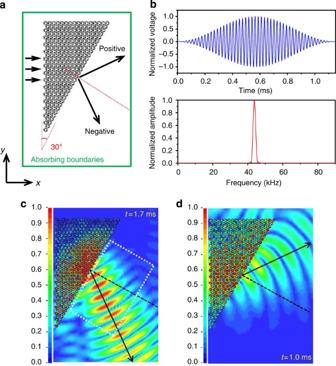Figure 3: Numerical simulation of transient wave propagation in a 2D medium containing the EMM. (a) Schematic of the transient simulation. A 30° prism-shaped EMM consisting of 256 unit cells is hosted in the steel plate with absorbing boundaries (green bounding box). An incident longitudinal wave is launched from the left, arriving normal to the vertical interface between the steel and the EMM prism. The refracted waves at the oblique interface are anticipated on the negative or positive side with respective to the surface normal (red dotted line). (b) Waveform (top) and frequency spectrum (bottom) of the tone-burst signal. (c) Amplitudes of the in-plane velocity fields atfc=43.8 kHz. The white dashed box indicates the region where the 2D spatial Fourier transform is applied. (d) Amplitudes of the in-plane velocity fields atfc=30 kHz. Figure 3c shows a snapshot of the normalized amplitude of the in-plane velocity field at f c =43.8 kHz and t =1.7 ms. At this frequency, E eff and ρ eff are calculated as −3.6 GPa and −5,891 kg m −3 , respectively. To quantitatively determine the angle of refraction, the 2D spatial Fourier transform is applied to the velocity field in the selected area in Fig. 3c . The angle of refraction is determined from the obtained velocity field in the 2D wavenumber domain ( k x −k y ). On the basis of the velocity field in the wavenumber domain ( k x −k y ), we can easily separate the refracted longitudinal and transverse waves. The angle of refraction, which is determined by the wave vector, can be estimated at the maximum normalized velocity amplitude as arctan( k y / k x )+30°. It is noticed that uncertainty exists for the angle of refraction due to uncertain area estimation of the maximum normalized velocity amplitude in the wavenumber domain. Therefore, the angle of wave refraction is estimated as −37.5±1° for frequency f c =43.8 kHz. The backward-wave propagation in the EMM is also evidenced by carefully comparing the transient wave propagation at different time steps from Supplementary Movie 1 . For comparison purposes, the snapshot of amplitude of in-plane velocity field at f c =30 kHz and t =1.0 ms is also illustrated in Fig. 3c . As expected, the refracted wave is located on the positive refraction area because the E eff and ρ eff are 30.8 GPa and 12,400 kg m −3 , respectively, and the forward-wave propagation in the EMM is also identified. Figure 3: Numerical simulation of transient wave propagation in a 2D medium containing the EMM. ( a ) Schematic of the transient simulation. A 30° prism-shaped EMM consisting of 256 unit cells is hosted in the steel plate with absorbing boundaries (green bounding box). An incident longitudinal wave is launched from the left, arriving normal to the vertical interface between the steel and the EMM prism. The refracted waves at the oblique interface are anticipated on the negative or positive side with respective to the surface normal (red dotted line). ( b ) Waveform (top) and frequency spectrum (bottom) of the tone-burst signal. ( c ) Amplitudes of the in-plane velocity fields at f c =43.8 kHz. The white dashed box indicates the region where the 2D spatial Fourier transform is applied. ( d ) Amplitudes of the in-plane velocity fields at f c =30 kHz. Full size image A prism-shaped EMM plate (326 mm × 192 mm × 1.5 mm) is then fabricated in a thin stainless steel (Grade 304) plate by using a precision laser cutting system, as shown in Fig. 4a . Zoomed-in views of the specimen at different scale bars are shown in Fig. 4b,c . In the design, the dimensions of the host plate are (3,048 mm × 1,829 mm × 1.5 mm) to eliminate any unwanted reflected waves from the boundaries. The geometrical parameters of the unit cell can be found in Table 1 . Since the interesting frequencies in this study are in a very low-frequency range (<50 kHz), the lowest symmetric Lamb wave mode (S 0 ) can be a good approximation for the longitudinal elastic wave in bulk stainless steels. 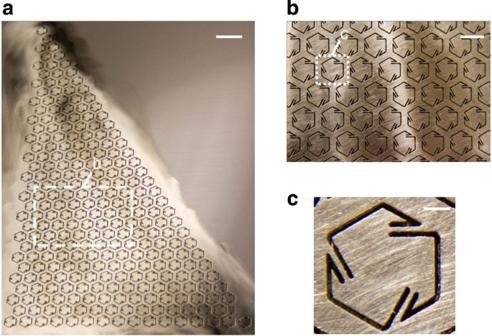Figure 4: Fabricated EMM sample. (a) The fabricated triangular array of the EMM. Scale bar, 20 mm. (b) Zoomed unit cells. Scale bar, 10 mm. (c) Zoomed single unit cell. Scale bar, 2 mm. Figure 4: Fabricated EMM sample. ( a ) The fabricated triangular array of the EMM. Scale bar, 20 mm. ( b ) Zoomed unit cells. Scale bar, 10 mm. ( c ) Zoomed single unit cell. Scale bar, 2 mm. Full size image The experimental set-up of the transient wave propagation in the EMM plate is shown in Fig. 5a . The in-plane longitudinal wave will be generated by using piezoelectric lead zirconate titanate (PZT) actuators. The in-plane time-dependent surface velocities are measured on the surface of the plate by a 3D laser scanning vibrometer (Polytec PSV-400-3D) based on the Doppler frequency-shift effect on light waves [33] . 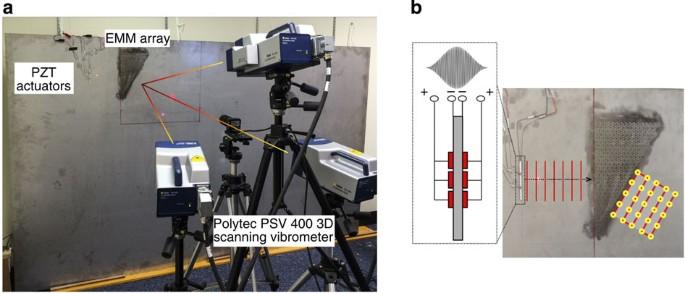Figure 5: Experimental measurement of the transient wave propagation in the EMM plate. (a) The experimental set-up of the transient wave propagation by using PZT actuators and 3D laser vibrometer. (b) Wave beam generation and measurement. The schematic cross-section view of the PZT pairs (small red rectangles) symmetrically bonded on the surface of stainless steel plate (large grey rectangle) is shown on the left of the photo. The in-plane longitudinal wave is incident from the left side of the EMM prism. The red lines and yellow circles on the right side of the EMM schematically demonstrate the point-by-point scanned path by lasering the defined surface area of the sample plate. Figure 5b shows the schematic of wave beam generation and measurement. Six rectangular PZT actuators (33.00 mm × 4.00 mm × 0.76 mm, 850WFB, APC International) are symmetrically bonded on the two surfaces of the plate (three on top and three on bottom) to generate the longitudinal (S 0 ) wave [34] , shooting normally onto the vertical surface of the prism. The aforementioned 50-cycle narrow-band tone-burst voltage signal is driven by a function generator (Tektronix AFG3021) and amplified by a wideband power amplifier (Krohn-Hite 7602M) [35] . Two central frequencies 43.8 and 30 kHz are chosen for the NR and positive refraction, respectively, and two corresponding laser scanning areas are defined for the measurements guided by the numerical simulations. For example, for f c =43.8 kHz, the measured area (156 mm × 123 mm) is specified at the lower part of the refracted region as shown in Fig. 6a . To get good sensitivity and resolution, a grid density of 3 mm and a total of 2,226 scan points are chosen for the scanning process. To measure the positively refracted waves with f c =30 kHz, the scanning area (189 mm × 123 mm) is located in the upper part of the refracted region. To ensure the signal quality, reflective spray is applied on the plate to enhance the surface reflection [36] and the measurement at each scan point is averaged 10 times. Enough waiting time is given between each measurement to ensure the plate ‘calms down’. The frequency–wavenumber filter technique [37] is also applied to remove undesired out-of-plane mode, which is generated due to the slight position mismatch of the actuator pairs. Figure 5: Experimental measurement of the transient wave propagation in the EMM plate. ( a ) The experimental set-up of the transient wave propagation by using PZT actuators and 3D laser vibrometer. ( b ) Wave beam generation and measurement. The schematic cross-section view of the PZT pairs (small red rectangles) symmetrically bonded on the surface of stainless steel plate (large grey rectangle) is shown on the left of the photo. The in-plane longitudinal wave is incident from the left side of the EMM prism. The red lines and yellow circles on the right side of the EMM schematically demonstrate the point-by-point scanned path by lasering the defined surface area of the sample plate. 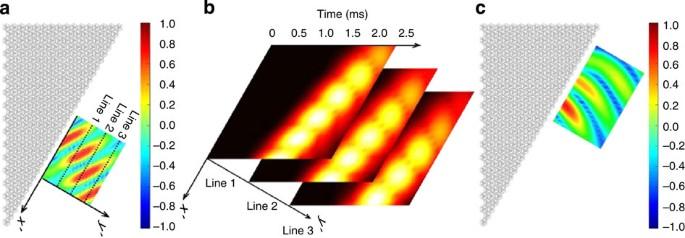Figure 6: Results of experimental measurements. (a) The measured in-plane velocity field att=1.7 ms whenfc=43.8 kHz. (b) Time-domain signal envelopes of the measured in-plane velocity on the three selected lines ina. (c) The measured in-plane velocity field att=1.0 ms whenfc=30 kHz. Full size image Figure 6: Results of experimental measurements. ( a ) The measured in-plane velocity field at t =1.7 ms when f c =43.8 kHz. ( b ) Time-domain signal envelopes of the measured in-plane velocity on the three selected lines in a . ( c ) The measured in-plane velocity field at t =1.0 ms when f c =30 kHz. Full size image For f c =43.8 kHz, the snapshot of normalized amplitude of the measured in-plane velocity field in the defined area at t =1.7 ms is shown in Fig. 6a . A local coordinate system x ′− y ′ is defined with x ′ parallel to the oblique interface. After applying the frequency–wavenumber filter technique to the received signals on each grid of the scanning area, any unwanted off-centre frequency components and out-of-plane wave modes are removed leaving only in-plane wave modes with a narrow band around f c . Therefore, comparing with the refracted velocity field from the numerical simulation as shown in Fig. 3a , a very good agreement between the experimental results and the simulation results can be observed. It can be clearly found that the refracted wave propagates downwards along the NR side with respect to the interface normal. By transforming the measured wave field from spatial domain to wavenumber domain, the angle of refraction can be obtained as 38±1°, which is very close to the numerical prediction (37.5±1°), even though losses are not taken into account in the numerical simulation. The uncertainty is determined from choosing a proper area covering the maximum normalized amplitudes of the measured velocity fields in the 2D wavenumber domain ( k x − k y ), which are obtained by conducting the 2D spatial Fourier transform to the snapshot of the experimentally measured velocity fields. Figure 6b shows the amplitudes of recorded wave signal envelopes in the time domain at three regularly spaced lines with a distance from one another of 33 mm along the y ′ direction (see inset in Fig. 6a —lines 1, 2 and 3). It is very convincing that the energy direction of the refracted wave beam is indeed on the NR side, and the wave pulses arrive at the three lines at different times with group velocity V g =3,320 m s −1 , which is the group velocity of the transverse wave. For f c =30 kHz, Fig. 6c shows the snapshot of the amplitude of the in-plane velocity field in the measured area at t =1.0 ms. Positive refraction is clearly identified at this central frequency, which is also in good agreement with the numerical prediction. It should be mentioned that the ordered configuration of the unit cells in the prism is chosen only for the simplicity of the design and fabrication. The double-negative effect is caused by the simultaneous translational and rotational resonances due to the interior chiral structures, as demonstrated in the Fig. 1b,c . In principle, the interior resonant mechanism is the same even for the EMM with random configuration of cells. For the proposed EMM, the inherently resonant structures interact with the elastic wave, but their size is much smaller than the wavelength in the host medium. Therefore, the sensitivity of NR to sample imperfections is very low and NR could still be found in the EMM with a random configuration of cells. Wave mode analysis of refracted waves Because of the vector nature of elastic waves, both longitudinal and transverse refracted wave components could be generated at the interface between the EMM and stainless steel. However, wave mode analysis of the negatively refracted waves has not yet been properly investigated due to the interference of the longitudinal and transverse waves, especially in the near field. To precisely explore the refracted wave modes and understand how the incident longitudinal wave will propagate through the EMM with chiral microstructure, EFCs of the EMM in the frequency range of 39–44.6 kHz in the first Brillouin zone are plotted in Fig. 7a . V g and k are the group velocity and wave vector in the EMM, respectively. V gt and k t are the group velocity and wave vector of the transverse wave in the host medium, respectively. The black dashed line represents the surface normal to the interface, which only crosses through the green dashed circle (transverse wave). First, it can be found that inside the EMM the group velocity and the phase velocity are opposite in direction since the EFCs decrease with increasing frequency. In addition, due to the anisotropy of the chiral microstructure, the EFC at the frequency does not possess the circular shape and displays a chiral pattern [32] . Second, based on the conservation of the component of the wave vector parallel to the refracted surface, the NR in the host medium is clearly demonstrated. The angle of the refracted transverse wave can be determined as ϕ =−37°, which is consistent with the angle experimentally measured in Fig. 6a , and no refracted longitudinal waves can be generated. That means that a wave mode conversion from the longitudinal waves to the transverse waves has occurred on the output surface of the metamaterial wedge owing to the double-negative effective material properties of the EMM at this frequency. 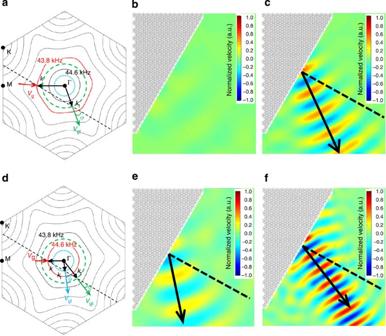Figure 7: Wave mode conversion at different excitation frequencies. (a) The EFCs of the EMM, transverse (green dashed circle) and longitudinal (blue dot circle) waves in stainless steel at 43.8 kHz. The EFC of the EMM at 43.8 kHz is highlighted with red solid curve. (b) The divergence of the velocity fields atfc=43.8 kHz. (c) The curl of the velocity fields atfc=43.8 kHz. (d) The EFCs of the EMM, transverse (green dashed circle) and longitudinal (blue dot circle) waves in stainless steel at 44.6 kHz. The EFC of the EMM at 44.6 kHz is highlighted with red solid curve. (e) The divergence of the velocity fields atfc=44.6 kHz. (f) The curl of the velocity fields atfc=44.6 kHz. Ina,d, the black dashed line represents the surface normal to the interface. Inb,c,e,f, the colour bar indicated the normalized amplitude of the velocity field. Figure 7: Wave mode conversion at different excitation frequencies. ( a ) The EFCs of the EMM, transverse (green dashed circle) and longitudinal (blue dot circle) waves in stainless steel at 43.8 kHz. The EFC of the EMM at 43.8 kHz is highlighted with red solid curve. ( b ) The divergence of the velocity fields at f c =43.8 kHz. ( c ) The curl of the velocity fields at f c =43.8 kHz. ( d ) The EFCs of the EMM, transverse (green dashed circle) and longitudinal (blue dot circle) waves in stainless steel at 44.6 kHz. The EFC of the EMM at 44.6 kHz is highlighted with red solid curve. ( e ) The divergence of the velocity fields at f c =44.6 kHz. ( f ) The curl of the velocity fields at f c =44.6 kHz. In a , d , the black dashed line represents the surface normal to the interface. In b , c , e , f , the colour bar indicated the normalized amplitude of the velocity field. Full size image To validate the wave mode conversion phenomenon, the divergence and curl of the refracted wave velocity fields are numerically calculated, as shown in Fig. 7b,c , which represent the longitudinal and transverse wave components, respectively. The velocity amplitudes in the two figures are normalized with the same amplitude value. A very weak refracted wave field can be found in the longitudinal wave mode, while a much stronger refracted wave field can be observed in the transverse wave mode. To demonstrate the conversion efficiency of the refracted transverse wave, the ratio between the input power of the incident longitudinal wave and the output power of the negatively refracted transverse wave has been calculated. In the calculation, the power flows of both the incident longitudinal wave and the refracted transverse wave are considered, which can be described by the Poynting vector P as (ref. 38 ), where v * is the complex conjugate of the particle velocity vector and σ is the stress field tensor. The power flow through a specified surface with the surface normal n can be calculated as P n = P · n . In our transient simulations, the input power of the incident longitudinal wave, , should be calculated by taking the spatial integral over the vertical surface of the prism, A v , and the time integral over a time range, Δ t , which is chosen to be long enough to cover the 50-cycle tone-burst signal as . Similarly, the output power of the refracted transverse wave, , should be calculated by taking the spatial integral over the oblique interface of the prism, A o , and the time integral over Δ t as . Then, the conversion efficiency of the refracted transverse wave can be defined as . At f c =43.8 kHz, we obtain the conversion efficiency c L−T =46.6% based on the transient simulation result. Notice that part of the input power transfers to the power of the reflected waves inside the EMM prism. Unlike the wave mode conversion between two conventional bulk media that can only be observed in the area of the positive refraction, the mode conversion of the refracted wave by using the double-negative EMM with chiral microstructure occurs in the area of the NR. Moreover, the behaviour of wave mode conversion in NR is mainly manipulated by the double-negative effective material properties of the EMM, therefore the wave mode conversion could be highly designable and tunable by carefully selecting or actively tuning the chiral structures (for example, through shunted piezoelectric patches) [39] . The condition of a complete mode conversion has been explicitly derived for the EMM with double-negative properties [29] , which cannot be accomplished in a conventional positive elastic medium. To illustrate the co-existed refracted longitudinal and transverse wave modes, the analysis of EFCs of the EMM and the host medium at frequency 44.6 kHz is also conducted in Fig. 7d . V gl and k l are group velocity and wave vector of the longitudinal wave in the host medium, respectively. The almost circular shape of the red EFC indicates that the EMM is effectively isotropic at higher frequency range. Similarly, by applying the Snell–Descartes law, NR for both the longitudinal wave and transverse wave can be identified at the frequency, and the angles of longitudinal refraction and transverse refraction can be obtained as ϕ =−23° and ψ =−50°, respectively. To separate the longitudinal and transverse waves, the divergence and curl of the refracted wave fields are also calculated in Fig. 7e,f , respectively. It can be found that the amplitude of the wave field in Fig. 7e is comparable to that in Fig. 7f , which means that the refracted wave mode conversion is not very significant when the incident wave frequency is larger than 44.2 kHz. Furthermore, to quantitatively investigate the wave mode conversion for NR as a frequency-dependant phenomenon, a frequency scan is conducted on the central frequency of the transient simulation. According to the EFC analysis, in the current system with angle of incidence fixed at 30°, the frequency ranges of NR are 43.0–45.0 kHz and 44.25–45.0 kHz for the longitudinal and transverse waves, respectively. On the basis of the results of the EFC analysis, we select the frequency scanning ranges for the transient simulations accordingly. The refracted longitudinal and transverse wave fields are separated by calculating the divergence and curl of the obtained velocity fields from the transient simulation at different central frequencies. The 2D spatial Fourier transform is then applied to the separated wave fields, and the normalized velocity amplitude profiles of the refracted waves in the wavenumber domain can be extracted at each central frequency. The normalized velocity amplitude profiles of the refracted transverse and longitudinal waves are plotted as functions of the frequency as shown in Fig. 8a,b , respectively. In the figures, the white line joins the points with maximum amplitude at different frequency points and therefore represents the frequency dependence of the angle of refraction for the given incident angle. 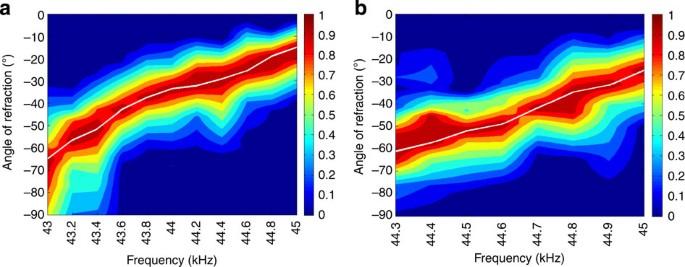Figure 8: Normalized velocity amplitude profiles as functions of frequency. (a) The normalized velocity amplitude profile of the refracted transverse wave mode. (b) The normalized velocity amplitude profile of the refracted longitudinal wave mode. Figure 8: Normalized velocity amplitude profiles as functions of frequency. ( a ) The normalized velocity amplitude profile of the refracted transverse wave mode. ( b ) The normalized velocity amplitude profile of the refracted longitudinal wave mode. Full size image In this article, we have designed and studied a single-phase EMM with chiral microstructure. Both the homogenization model and the band structure calculation show the existence of a negative band for elastic waves in a large subwavelength frequency range (41.8–45.0 kHz), which is produced simultaneously by translational and rotational resonances. The proposed EMM is then manufactured and the experimental work is implemented on the fabricated EMM plate to demonstrate the NR phenomenon. The negatively and positively refracted wave fields over a certain time range in selected regions are measured by using a scanning laser vibrometer. The experimentally estimated NR angles are in good agreement with the numerical simulations. Accompanying NR, we also discuss the refracted wave mode conversion, which again supports our analysis and experimental results on NR of an elastic wave by the EMM with chiral microstructure. The proposed EMM with the unit cell size close to a tenth of a wavelength extends the research of elastic wave control in the deep-subwavelength scale and may bring potential breakthrough for the engineering applications in manipulation of in-plane waves, in-plane-guided wave cloaking, super-resolution wave sensors by integrating the EMM into the plate structure, in-plane wave superlens and structural health monitoring in aerospace plate structures. How to cite this article : Zhu, R. et al. Negative refraction of elastic waves at the deep-subwavelength scale in a single-phase metamaterial. Nat. Commun. 5:5510 doi: 10.1038/ncomms6510 (2014).